A molecule-like PtAu24(SC6H13)18nanocluster as an electrocatalyst for hydrogen production The theoretically predicted volcano plot for hydrogen production shows the best catalyst as the one that ensures that the hydrogen binding step is thermodynamically neutral. However, the experimental realization of this concept has suffered from the inherent surface heterogeneity of solid catalysts. It is even more challenging for molecular catalysts because of their complex chemical environment. Here, we report that the thermoneutral catalyst can be prepared by simple doping of a platinum atom into a molecule-like gold nanocluster. The catalytic activity of the resulting bimetallic nanocluster, PtAu 24 (SC 6 H 13 ) 18 , for the hydrogen production is found to be significantly higher than reported catalysts. It is even better than the benchmarking platinum catalyst. The molecule-like bimetallic nanocluster represents a class of catalysts that bridge homogeneous and heterogeneous catalysis and may provide a platform for the discovery of finely optimized catalysts. Hydrogen (H 2 ) has been considered as an alternative energy carrier and generated the intense interest in creating artificial catalytic systems that can efficiently produce H 2 from water [1] , [2] , [3] , [4] . Hydrogenase enzymes that contain iron and nickel cofactors are efficient hydrogen evolution reaction (HER) catalysts with turnover frequencies (TOFs) as high as 9,000 mol of H 2 per mole of catalyst per second (mol H 2 (mol cat) −1 s −1 ) [5] . There have been a variety of synthetic molecular catalysts, including nickel, cobalt, iron and molybdenum complexes, to mimic the biological catalysts [6] , [7] , [8] , [9] , [10] , [11] , [12] . However, the TOF values reported for these complexes remain quite low (<4.1 mol H 2 (mol cat) −1 s −1 ), and they often show limited stability in aqueous media [13] . Moreover, practical electrocatalysis typically requires their immobilization on electrode materials that can operate fully in aqueous media [14] , [15] . Recent progress in the computational design of solid catalysts has revealed the importance of engineering of the structure and adsorption energies for catalysis at surfaces [16] , [17] , [18] . In fact, some engineered surface alloys exhibit high catalytic activities comparable to platinum [18] . However, the inherent heterogeneity in the surface structure and composition often found in these solid catalysts hamper the fine controlling of these properties at the molecular scale. Ligand-protected gold and silver nanoclusters have received much attention as materials with many practical applications because of promises offered by their unique optical, electrochemical and catalytic properties [19] , [20] , [21] , [22] . Unlike the supported cluster systems [23] , [24] , these clusters are stable without the support and readily soluble in appropriate solvents. They have special stability at certain compositions, and thus molecule-like clusters with precise compositions are typically obtained from various size-controlled syntheses [21] , [22] . Au 25 (SR) 18 , Au 102 (SR) 44 and Ag 44 (SR) 30 , where SR is a thiolate ligand, are the examples of these clusters whose stability is thought to arise from the closure of superatomic electron shells [25] , [26] , [27] . While stable clusters to date are rather limited to Au and Ag systems, bimetallic clusters prepared by doping a foreign metal into the stable Au and Ag clusters have opened an avenue to the fine-tuning of the cluster properties [28] , [29] , [30] , [31] , [32] , [33] . Here we report a highly active HER catalyst based on a molecule-like bimetallic cluster that can generate H 2 with TOFs of 4.8 in tetrahydrofuran (THF) and 34 mol H 2 (mol cat) −1 s −1 in water, respectively, at a moderate overpotential ( η =0.6 V). This cluster catalyst represents a special type of catalyst that bridges homogeneous and heterogeneous catalysis. Molecule-like metal nanoclusters It has been found that Pt can selectively replace the central gold atom in the Au 25 cluster, leading to a single Pt-doped bimetallic cluster ( Fig. 1a ) [30] , [33] , [34] . The Au 25 and Pt-doped clusters were synthesized according to the procedures reported elsewhere [34] (see Supplementary Notes 1–3 for details). Although they have been fully characterized in our previous report [34] , we will next briefly discuss their mass spectra, and optical and electrochemical properties, which can serve as an introduction to these molecule-like metal clusters. In Fig. 1b , the matrix-assisted laser desorption ionization mass spectra of the isolated gold (red) and Pt-doped gold clusters (blue) show only a single peak, indicating that the isolated clusters are extremely monodisperse. The peak at m / z ∼ 7,034 Da observed for the gold cluster (red) corresponds to the intact ion with a chemical composition of Au 25 (SC 6 H 13 ) 18 . The peak at m/z ∼ 7,032 Da observed for the Pt-doped gold cluster is however almost superimposed with that of Au 25 (SC 6 H 13 ) 18 due to their small mass difference. The isotope pattern of the Pt-doped gold cluster (blue) shown in the inset of Fig. 1b can clearly be distinguished from that of Au 25 (SC 6 H 13 ) 18 (red) and matches well with the simulated isotope pattern (black) of PtAu 24 (SC 6 H 13 ) 18 , manifesting that one Au atom in the Au 25 cluster has been cleanly replaced by a Pt atom. Hereafter, these clusters will be abbreviated as Au 25 and PtAu 24 , respectively. The average core size of both clusters is found to be around 1.1 nm ( Supplementary Fig. 1 ). 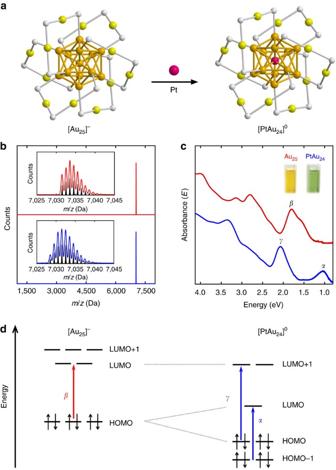Figure 1: Characterizations of molecule-like metal clusters. (a) Structures of Au25and PtAu24clusters (golden, gold atoms of the core; olive, gold atoms of the shell; grey, sulfur (the rest of the ligand is omitted for clarity)). (b) Matrix-assisted laser desorption ionization (MALDI) mass spectra of Au25(SC6H13)18(red) and PtAu24(SC6H13)18(blue). The insets show the comparisons between the experimental data and the simulated isotope patterns (black sticks). (c) UV-vis-NIR absorption spectra of [Au25]−(red) and [PtAu24]0(blue) in tetrachloroethylene. The wavelength-scale absorption spectrum, Abs(λ), was converted to the energy-scale spectrum, absorbance (E), according to the relation Abs(E)∝[Abs(λ)]λ2. The insets show the photographs of [Au25]−and [PtAu24]0in CH2Cl2. (d) Electronic energy levels of [Au25]−and [PtAu24]0.α,βandγdenote the optical transitions observed for [Au25]−and [PtAu24]0inc. Figure 1: Characterizations of molecule-like metal clusters. ( a ) Structures of Au 25 and PtAu 24 clusters (golden, gold atoms of the core; olive, gold atoms of the shell; grey, sulfur (the rest of the ligand is omitted for clarity)). ( b ) Matrix-assisted laser desorption ionization (MALDI) mass spectra of Au 25 (SC 6 H 13 ) 18 (red) and PtAu 24 (SC 6 H 13 ) 18 (blue). The insets show the comparisons between the experimental data and the simulated isotope patterns (black sticks). ( c ) UV-vis-NIR absorption spectra of [Au 25 ] − (red) and [PtAu 24 ] 0 (blue) in tetrachloroethylene. The wavelength-scale absorption spectrum, Abs( λ ), was converted to the energy-scale spectrum, absorbance ( E ), according to the relation Abs( E ) ∝ [Abs( λ )] λ 2 . The insets show the photographs of [Au 25 ] − and [PtAu 24 ] 0 in CH 2 Cl 2 . ( d ) Electronic energy levels of [Au 25 ] − and [PtAu 24 ] 0 . α , β and γ denote the optical transitions observed for [Au 25 ] − and [PtAu 24 ] 0 in c . Full size image The ultraviolet-vis-near-infrared (NIR) absorption spectra in Fig. 1c show distinctively different profiles of Au 25 and PtAu 24 clusters. The absorption profile is shown in the photon energy scale to show the broad NIR peak more clearly. The Au 25 cluster exhibits the characteristic absorption features of Au 25 clusters with peaks at 1.8, 2.8 and 3.1 eV. On Pt doping, the absorption profile changes drastically; that is, there is a new absorption band that appears at 2.1 eV with an additional NIR band centred at 1.1 eV in the low-energy region. The absorption profile of the Pt-doped cluster is consistent with that of neutral [PtAu 24 ] 0 where the Pt dopant is located at the centre of the core [33] . Evidently, replacing the central Au atom with Pt results in stable [PtAu 24 ] 0 having a superatomic 6-electron configuration [25] , [26] , [34] . The change in superatomic electronic configuration from 8-electron [Au 25 ] − to 6-electron [PtAu 24 ] 0 would lead to the splitting of the 1P orbital accompanying a Jahn–Teller-like distortion of the PtAu 12 core [34] . The appearance of the new bands at 1.1 eV ( α ) and 2.1 eV ( γ ) and the disappearance of the band at 1.8 eV ( β ) for [PtAu 24 ] 0 in Fig. 1c,d are the results of the change in electronic structure of PtAu 24 . Electrochemistry and electrocatalytic activities The optical measurements show that the electronic structure of Au 25 cluster is drastically altered on doping of a Pt atom. To further unravel the electronic structure of the PtAu 24 cluster, square-wave voltammetry (SWV) of Au 25 and PtAu 24 clusters were conducted. Voltammetry has been effectively used to study the electron transfer properties and the electronic structures of gold nanoclusters [19] , [34] . Understanding the redox behaviours near the HOMO-LUMO (highest occupied and lowest unoccupied molecular orbitals) levels is of particular importance in the design of efficient electrocatalysts. The SWVs in Fig. 2a exhibit well-resolved current peaks that lie at the formal potentials of the cluster charge-state couples. The open-circuit potential was found at −0.49 V for the Au 25 cluster, indicating that the Au 25 cluster is in anionic form, that is, [Au 25 ] − . Therefore, the current peaks observed at −0.39 (O1), −0.04 (O2) and 0.69 (O3) correspond to the first, second and third oxidation peaks of the [Au 25 ] − cluster, while the peak at −2.06 V (R1) corresponds to the first reduction peak. The electrochemical gap determined from the difference between the first oxidation (O1) and reduction (R1) potentials is found to be 1.67 V. The HOMO-LUMO gap for [Au 25 ] − is determined to be 1.32 V by subtracting the charging energy term (O1–O2) of 0.35 V from the O1–R1 gap. 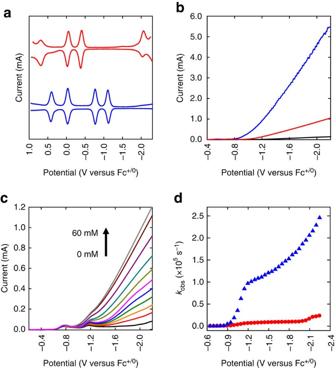Figure 2: Voltammograms and electrocatalytic activities of metal clusters. (a) SWVs of Au25(red) and PtAu24(blue) in CH2Cl2(0.1 M Bu4NPF6). (b) LSVs in THF (0.1 M Bu4NPF6) solution containing 1.0 M TFA in the absence (black) and presence of 1 mM Au25(red) and 1 mM PtAu24(blue) at 50 mVs−1. (c) LSVs of PtAu24(1 mM) in THF (0.1 M Bu4NPF6) at 50 mVs−1in the presence of 0, 4, 8, 12, 17, 21, 27, 34, 45, 55 and 60 mM of TFA. (d)kobs-potential plots for Au25(red) and PtAu24(blue) in the presence of 1.0 M TFA. For the precise comparison, measured potentials were corrected using ferrocene (Fc+/0) as an internal standard. Figure 2: Voltammograms and electrocatalytic activities of metal clusters. ( a ) SWVs of Au 25 (red) and PtAu 24 (blue) in CH 2 Cl 2 (0.1 M Bu 4 NPF 6 ). ( b ) LSVs in THF (0.1 M Bu 4 NPF 6 ) solution containing 1.0 M TFA in the absence (black) and presence of 1 mM Au 25 (red) and 1 mM PtAu 24 (blue) at 50 mVs −1 . ( c ) LSVs of PtAu 24 (1 mM) in THF (0.1 M Bu 4 NPF 6 ) at 50 mVs −1 in the presence of 0, 4, 8, 12, 17, 21, 27, 34, 45, 55 and 60 mM of TFA. ( d ) k obs -potential plots for Au 25 (red) and PtAu 24 (blue) in the presence of 1.0 M TFA. For the precise comparison, measured potentials were corrected using ferrocene (Fc +/0 ) as an internal standard. Full size image The redox potentials are drastically altered on doping of a Pt atom in the core as can be seen in Fig. 2a . Unlike the anionic Au 25 cluster, PtAu 24 is charge neutral with the open-circuit potential found at −0.49 V. Thus, the current peaks observed at −0.03 (O1) and 0.41 (O2) correspond to the first and second oxidation peaks of the PtAu 24 cluster, while −0.76 (R1) and −1.10 V (R2) correspond to the first and second reduction peaks. The observed O1–R1 gap and the deduced HOMO-LUMO gaps from the SWV in Fig. 2a are found to be dramatically reduced to 0.73 V and 0.29 V, respectively. This result indicates that the electronic structure has indeed been greatly altered on Pt doping, and, more importantly, reduction potentials of [PtAu 24 ] 0 shifted positively by nearly 1 V compared to that of [Au 25 ] − , potentially offering the possibility to lower overpotentials for reductive electrocatalysis. Figure 2b shows linear sweep voltammograms (LSVs) in THF (0.1 M Bu 4 NPF 6 ) solution containing 1.0 M trifluoroacetic acid (TFA) in the absence (black) and presence of Au 25 (red) and PtAu 24 (blue) clusters at a glassy carbon electrode (GCE). Compared to the blank current, the current for the proton reduction is significantly increased in the presence of Au 25 . The current further increases in the presence of PtAu 24 . The onset potential ( E onset ) of catalytic current is observed at −1.10 V for Au 25 , positively shifted by 150 mV compared to that of the blank GCE. In the presence of PtAu 24 , the onset was found at −0.89 V, positively shifted by 360 mV. The thermodynamic reduction potential of proton is estimated to be −0.82 V in THF (1.0 M TFA) and thus the onset potential of −0.89 observed for PtAu 24 corresponds to an overpotential of 70 mV (refs 35 , 36 ), which is comparable to that of natural hydrogenase ( ∼ 100 mV) enzymes [37] . The catalytic activity of PtAu 24 was further examined with increasing the concentration of TFA. As shown in Fig. 2c , the LSV clearly shows current peaks at −0.76 and −1.10 V corresponding to the first and second reduction of the PtAu 24 cluster. Whereas there is no significant change observed for the [PtAu 24 ] 0/− peak, the [PtAu 24 ] −/2− peak current drastically increases with TFA, suggesting that HER is greatly enhanced at the potential where [PtAu 24 ] 2− is formed. That the HER current increases at the potential of the [PtAu 24 ] −/2− couple strongly suggests that PtAu 24 acts as an electron transfer mediator for HER that shuttles electrons from GCE to proton in the solution [38] , [39] . Interestingly, the onset potential of the second reduction of PtAu 24 matches well with the E onset (−0.89 V) observed in Fig. 2b , suggesting that the HER catalytic activity is indeed dependent on the charge state of PtAu 24 . When the catalytic activity of Au 25 was examined with increasing concentration of TFA, the current increase at a more negative potential (−1.1 V) and the reduction current associated with HER was found to be much smaller ( Supplementary Fig. 2 ). This result unambiguously shows that Pt doping significantly alters the redox potentials of the host cluster and thus drastically enhance its catalytic activity. In addition, the charge-state-dependent catalytic activity of PtAu 24 clusters indicates that they are like molecular catalysts that carry discrete charge for reaction, which sets these clusters apart from other metal nanoparticle systems. At sufficiently high acid concentration relative to the catalyst, the following equation can be used to calculate pseudo-first-order rate constant, k obs , for H 2 evolution that is catalysed by freely diffusing catalysts: [6] , [13] , [40] where I c is the catalytic current, I p is the peak current in the absence of acid (here taken from the wave of [PtAu 24 ] 0/− or [Au 25 ] 0/− ), 2 is the number of electrons involved in the catalytic reaction, R is the ideal gas constant, T is the temperature in Kelvin, F is Faraday’s constant and v is the scan rate. As can be seen in Supplementary Fig. 3a , I c increases with increasing acid concentration and levels off above 1.0 M TFA. At the acid concentration of 1.0 M, k obs was then obtained by plotting I c / I p as a function of v −1/2 as shown in Supplementary Fig. 3b . The k obs value calculated from the slope of the fit line ( Supplementary Fig. 3b ) is 121,000 s −1 at −1.5 V ( η =650 mV). Under the same experimental condition, the k obs value calculated in the presence of Au 25 is only 8,000 s −1 . The rate constant observed for PtAu 24 is also significantly higher than those reported to date for highly active molecular electrocatalysts; compared to cobalt complexes (700 s −1 at η =890 mV) [41] and copper complexes (11,000 s −1 at η =720 mV) [13] in comparable conditions, it is ca. 170- and 11-fold higher, respectively. To the best of our knowledge, the highest k obs value (106,000 s −1 ) thus far reported was observed at η =650 mV for a nickel complex that catalyses H 2 formation with pendant amines that act as proton relays [6] . The k obs value obtained for PtAu 24 is also higher than that. To understand the origin of the extraordinary catalytic activity observed for PtAu 24 , we compared k obs as a function of potential. As can be seen in Fig. 2d , the k obs value found at −0.89 V is 1,300 s −1 and sharply increases to 62,000 s −1 at −1.1 V, followed by a gradual increase to 186,000 s −1 at −2.0 V. Interestingly, the potential where the drastic increase occurs matches well with the second reduction wave [PtAu 24 ] −/2− . By contrast, the k obs value calculated for Au 25 is found to be relatively small (<16,000 s −1 ) until −2.1 V, where [Au 25 ] − is reduced to [Au 25 ] 2− . Mechanisms of HER The mechanism study shown in Fig. 3 clearly exhibits the charge-state-dependent catalytic activity of PtAu 24 . That is, the catalytic currents observed at potentials negative to the [PtAu 24 ] −/2− wave (that is, −1.3, −1.8 and −2.2 V) all exhibit linear correlation with [PtAu 24 ] and [TFA] 1/2 , respectively, which is consistent with the heterolytic HER mechanism (equation (3)) [42] , [43] . On the other hand, at −1.0 V where PtAu 24 is predominantly present in the form of [PtAu 24 ] − , the currents exhibit linear correlation with [TFA] and [PtAu 24 ] 3/2 , respectively, as shown in Fig. 3 insets, indicating the homolytic HER mechanism (equation (4)) [42] . 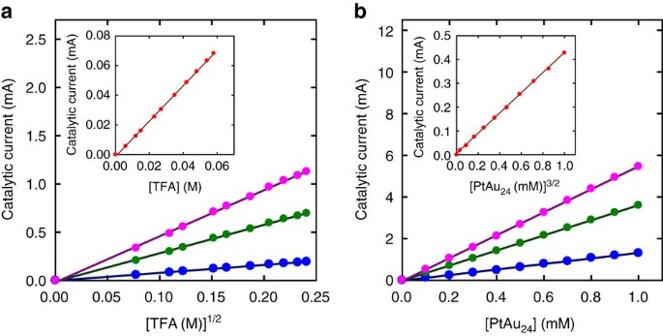Figure 3: Charge-state-dependent electrochemical HER mechanisms catalysed by PtAu24. Dependence of the catalytic current,Ic, (a) on the concentration of TFA in the presence of PtAu24(1 mM) and (b) on the concentration of PtAu24in TFA (1.0 M) solution at −1.3 (blue), −1.8 (green) and −2.2 V (purple). Insets show plots for dependence of theIcon the concentration of (a) TFA and (b) PtAu24at −1.0 V. The data are fitted by first-order linear functions (solid lines). Figure 3: Charge-state-dependent electrochemical HER mechanisms catalysed by PtAu 24 . Dependence of the catalytic current, I c , ( a ) on the concentration of TFA in the presence of PtAu 24 (1 mM) and ( b ) on the concentration of PtAu 24 in TFA (1.0 M) solution at −1.3 (blue), −1.8 (green) and −2.2 V (purple). Insets show plots for dependence of the I c on the concentration of ( a ) TFA and ( b ) PtAu 24 at −1.0 V. The data are fitted by first-order linear functions (solid lines). Full size image Heterolytic pathway: Homolytic pathway: This result is very reasonable considering the charge state of PtAu 24 . [PtAu 24 ] 2− reacts with proton to form [H-PtAu 24 ] − intermediate that is negatively charged and thus preferably react with proton to evolve H 2 . On the other hand, at −1.0 V [PtAu 24 ] − reacts with proton to form [H-PtAu 24 ] 0 intermediate that favours homolytic HER pathway. Similar charge-state dependence is observed for Au 25 . As shown in Supplementary Fig. 4 , the catalytic currents exhibit linear correlation with [TFA] and [Au 25 ] 3/2 , respectively, indicating homolytic pathway, at −1.0, −1.3 and −1.8 V, where Au 25 clusters are present in the form of [Au 25 ] − . When the cluster is reduced to [Au 25 ] 2− at −2.2 V, the currents exhibit linear correlation with [TFA] 1/2 and [Au 25 ], respectively, as shown in the insets of Supplementary Fig. 4 , indicating the heterolytic HER pathway. The charge-state-dependent catalytic activity has been observed for electrocatalysis using Co complexes where [Co(II)H] − favours heterolytic HER pathway, while homolytic pathway is favoured by [Co(III)H] 0 intermediate [44] . The charge-state-dependent catalytic activity of PtAu 24 observed in this work clearly display the characteristic of molecular catalysts. The charge state is not the only factor affecting the HER activity of the clusters. Comparing [PtAu 24 ] 2− with [Au 25 ] 2− , the k obs value calculated for [PtAu 24 ] 2− is 229,000 s −1 , more than 10-fold higher than that of [Au 25 ] 2− (22,000 s −1 ) at −2.2 V at which both clusters are present as a dianionic form. The vastly different catalytic activity can be understood by considering the reduction potential match between the catalyst and the substrate (proton). That is, when the reduction potential of catalyst matches closely with the thermodynamic potential of proton, the catalyst can act as an effective electron transfer mediator and enhance its activity dramatically [41] , [45] , [46] . In this work, the reduction potential of catalyst can be precisely tuned to match with the potential of HER by Pt doping, enabling judiciously optimized electrocatalysis. To gain further insight into the origin of the extraordinary catalytic activity of PtAu 24 , we have compared the hydrogen adsorption and the HER energetics calculated using density functional theory (DFT) for each cluster. We modelled the HER process by using protons solvated by two THF molecules, which are then adsorbed on the cluster surface; the whole system is further solvated by an implicit solvation model. 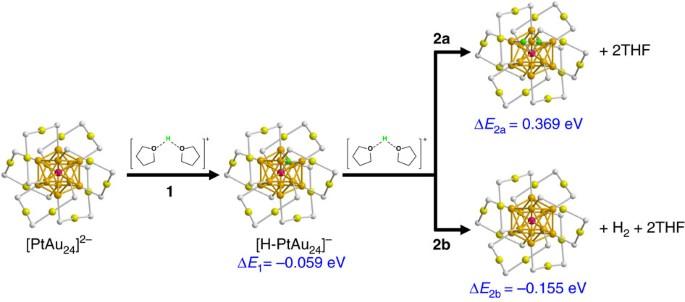Figure 4: Calculated reaction energies for H2evolution on PtAu24. In step 1, a solvated proton is transferred from THF molecules to [PtAu24]2−to form [H-PtAu24]−; in step 2a, a second solvated proton is transferred from THF molecules to [H-PtAu24]−to form [2H-PtAu24]; in step 2b, a second solvated proton reacts with H in [H-PtAu24]−to form H2. The calculations are at the DFT-TPSS level; besides the two explicit solvent molecules, an implicit solvent model is also included for the whole system (see ‘Methods’ section). Colour code for the cluster structure: golden, Au atoms of the core; olive, Au atoms of the shell; purple, Pt atom; green, adsorbed H from the liquid medium; grey, S (the rest of ligand is omitted for clarity). Figure 4 shows that the energy change of the Volmer step (step 1) calculated for [PtAu 24 ] 2− is rather thermodynamically neutral (−0.059 eV), whereas that for [Au 25 ] − is 0.539 eV. This result clearly suggests the initial hydrogen binding is energetically favourable on [PtAu 24 ] 2− , but is endothermic on [Au 25 ] − , explaining the high HER activity observed for [PtAu 24 ] 2− . However, the second H adsorption on [PtAu 24 ] 2− and [Au 25 ] − is found to be both endothermic; 0.369 and 1.21 eV for [H-PtAu 24 ] − (step 2a in Fig. 4) and [H-Au 25 ] 0 , respectively. Thus, the DFT calculations predict that hydrogen evolution occurs on PtAu 24 via the coupling of the adsorbed hydrogen with another proton from the solution (that is, heterolytic or Heyrovsky pathway) with an energy change of −0.155 eV (step 2b in Fig. 4). By contrast, the most thermodynamically favourable H 2 generation occurs on Au 25 via the homolytic pathway ( Supplementary Fig. 5 ). These calculation results are indeed in consistent with the experimentally found HER mechanisms for [PtAu 24 ] 2− and [Au 25 ] − . The idea of thermoneutral catalysts for HER regarding hydrogen binding has been demonstrated experimentally for pure metals, alloys and layered solid catalysts [16] , [17] , [18] , [47] . Recently, it has been pointed out that this concept can be applied to molecular complexes, although it is significantly difficult to find the thermoneutral complexes because of their inherently complex chemical environment [17] , [35] , [48] . In this work, we have demonstrated that the redox potentials and binding affinity can be fine-tuned by simple doping of a Pt atom into gold catalysts, opening a new avenue to the fine-tuning of the catalytic properties. Figure 4: Calculated reaction energies for H 2 evolution on PtAu 24 . In step 1, a solvated proton is transferred from THF molecules to [PtAu 24 ] 2− to form [H-PtAu 24 ] − ; in step 2a, a second solvated proton is transferred from THF molecules to [H-PtAu 24 ] − to form [2H-PtAu 24 ]; in step 2b, a second solvated proton reacts with H in [H-PtAu 24 ] − to form H 2 . The calculations are at the DFT-TPSS level; besides the two explicit solvent molecules, an implicit solvent model is also included for the whole system (see ‘Methods’ section). Colour code for the cluster structure: golden, Au atoms of the core; olive, Au atoms of the shell; purple, Pt atom; green, adsorbed H from the liquid medium; grey, S (the rest of ligand is omitted for clarity). Full size image Figure 4 also shows that the hydrogen preferably binds on the hollow site of the surface of the PtAu 12 core. It is interesting to note that the bond distance between the central Pt and the adsorbed H is found to be 1.788 Å, significantly shorter than the distance between the surface Au and the adsorbed H (2.031 Å), indicating that the adsorbed H atom forms H-Pt chemical bond with the central Pt. In the DFT calculations, we initially placed the H atom on the intact cluster surface away from the Au atoms; during geometry optimization, we found that the H atom spontaneously moves into the subsurface to interact directly with the central Pt atom while breaking some surface Au-Au bonds. This result suggests that the H-Pt bond formation is a downhill process with no transition state. The H-Pt bond is also manifested in the local electronic density of states ( Supplementary Fig. 6 ) that shows the hybridization between Pt 5 d states and the H 1 s state. The stronger H–Pt interaction than the H–Au interaction is a key factor contributing to the favourable HER energetics ( Fig. 4 ) on [PtAu 24 ] 2− than on [Au 25 ] − . Electrocatalytic H 2 production To verify the catalytic production of H 2 , we carried out controlled potential electrolysis (CPE) with PtAu 24 in THF containing 1.0 M TFA in an H-type cell. 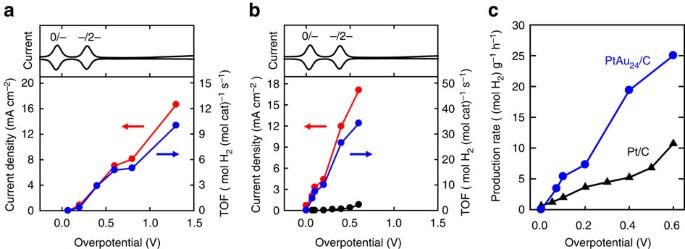Figure 5: CPE data for PtAu24in homogeneous and heterogeneous conditions. (a) Average current densities (red circles) and TOFs (blue circles) obtained at various overpotentials after 15 min homogeneous CPE in THF (0.5 M Bu4NPF6) containing 1.0 TFA with a glassy carbon plate (1 cm2) in the presence of PtAu24(2.5 μM). (b) Average current densities (red circles) and TOFs (blue circles) obtained at various overpotentials after 60 min heterogeneous CPE in 1.0 M Brinton–Robinson buffer solution (pH 3) on a PtAu24/C/GDL electrode (1 cm2). Average current densities obtained on a blank C/GDL (black circles) are shown for comparison. SWVs of PtAu24shown in the upper part of the graphs show the charge state of PtAu24at each overpotential. (c) H2production rates per mass of metals in the catalyst ((mol H2) g−1h−1) at various overpotentials on a PtAu24/C/GDL (blue circles) and a Pt/C/GDL (black triangles) electrodes (1 cm2). Figure 5a shows plots of the average current density and the amount of H 2 detected by gas chromatography analysis at each overpotential. The clusters display symptoms of decomposition after prolonged CPE experiments and thus the electrolysis was conducted for 15 min. As can be seen in the figure, production of H 2 is first detected at an overpotential of 0.2 V and increases with increasing overpotential. Comparison of the amount of H 2 produced with the charge consumed indicates that the current efficiency for H 2 production is > 97% when the overpotential is 0.4 V or higher. After subtracting the H 2 production from the blank solution, the TOF at η =0.6 V is found to be 4.8 mol H 2 (mol cat) −1 s −1 . To the best of our knowledge, this value is considerably higher than any other molecular catalysts reported for HER in similar conditions [6] , [7] , [8] , [9] , [12] , [13] . The highest TOF value reported thus far is 4.1 mol H 2 (mol cat) −1 s −1 obtained for a copper complex at a higher overpotential of 0.75 V (ref. 13 ). The nickel complex exhibiting a k obs value of 106,000 s −1 shows a TOF of 0.24 mol H 2 (mol cat) −1 s −1 at η =0.92 V (ref. 6 ). Figure 5: CPE data for PtAu 24 in homogeneous and heterogeneous conditions. ( a ) Average current densities (red circles) and TOFs (blue circles) obtained at various overpotentials after 15 min homogeneous CPE in THF (0.5 M Bu 4 NPF 6 ) containing 1.0 TFA with a glassy carbon plate (1 cm 2 ) in the presence of PtAu 24 (2.5 μM). ( b ) Average current densities (red circles) and TOFs (blue circles) obtained at various overpotentials after 60 min heterogeneous CPE in 1.0 M Brinton–Robinson buffer solution (pH 3) on a PtAu 24 /C/GDL electrode (1 cm 2 ). Average current densities obtained on a blank C/GDL (black circles) are shown for comparison. SWVs of PtAu 24 shown in the upper part of the graphs show the charge state of PtAu 24 at each overpotential. ( c ) H 2 production rates per mass of metals in the catalyst ((mol H 2 ) g −1 h −1 ) at various overpotentials on a PtAu 24 /C/GDL (blue circles) and a Pt/C/GDL (black triangles) electrodes (1 cm 2 ). Full size image While PtAu 24 exhibits high catalytic activity for H 2 production with moderate overpotential requirements in a non-aqueous solvent, it would be more practical if it can be immobilized on electrode materials that can fully operate in aqueous media. There are a number of immobilization strategies available for gold nanoparticles via their surface functionalization [39] , [49] , [50] . In this work, PtAu 24 cluster solution mixed with a carbon black (C) and Nafion was dropcast on a gas diffusion layer (GDL) electrode (PtAu 24 /C/GDL). We found that the clusters immobilized on the carbon black with the Nafion binder exhibit higher stability during electrolysis. Figure 5b shows plots of the average current density and the amount of H 2 detected after 60 min CPE at each overpotential in 1.0 M Brinton–Robinson buffer solution (pH 3). As can be seen in the figure, H 2 generation was achieved near the thermodynamic potential ( η =70 mV), which also matches very well with the E onset found in Fig. 2b . The charge passed and H 2 generation increased rapidly with increasing overpotential and the current efficiency for HER went up to nearly 100% when the overpotential is 100 mV or higher. At η =400 mV, the average current density increases above 12 mA cm −2 . Having immobilized such well-defined clusters on the electrode, we were able to calculate the TOF from the CPE experiments. As can be seen in Fig. 5b , the TOF values obtained from the heterogeneous catalysis are remarkably high; 34 mol H 2 (mol cat) −1 s −1 at η =0.6 V in aqueous media after subtracting the contribution from the blank C/GDL electrode. This value is again much higher than those obtained in comparable conditions. For comparison, a TOF of 2.2 mol H 2 (mol cat) −1 s −1 was obtained at η =0.59 V in acetate buffer (pH 4.5) for a cobalt catalyst immobilized on carbon nanotubes [14] . Although it is not straightforward to directly compare the TOF values obtained from the homogeneous ( Fig. 5a ) and heterogeneous ( Fig. 5b ) catalysis, the enhanced TOF obtained in the latter in aqueous media is highly encouraging and may reflect the fact that all clusters on the electrode are available for catalysis. The high catalytic activity observed for the PtAu 24 /C/GDL electrode has prompted us to compare its activity with the benchmarking Pt/C (commercial 20 wt% Pt on Vulcan carbon black) dropcast on a GDL electrode (1 cm 2 ). Since TOF could not be determined for the Pt/C, we have compared the H 2 production rate per mass of metals (that is, Au+Pt) in the catalyst composites (mol H 2 g −1 h −1 ). As can be seen in Fig. 5c , both PtAu 24 /C/GDL and Pt/C/GDL electrodes start to produce H 2 near the thermodynamic potential, but the H 2 production rate determined for the PtAu 24 /C/GDL is much higher than that for the Pt/C/GDL. For instance, the H 2 production rate determined for the PtAu 24 /C/GDL is 25 mol H 2 g −1 h −1 , which is more than two times higher than that for the Pt/C/GDL catalyst (11 mol H 2 g −1 h −1 ) at the same overpotential of 0.6 V. Here we show that the electronic structure and the catalytic activity of a cluster catalyst can be fine controlled by doping a Pt atom into a stable gold cluster. The bimetallic cluster is molecule-like and exhibits excellent catalytic activity for H 2 production; significantly higher than any other molecular catalysts reported thus far, to the best of our knowledge, and even higher than the benchmarking platinum catalyst. Mechanistic investigations have revealed that hydrogen binding step on the bimetallic cluster is thermodynamically neutral and the central Pt atom forms Pt-H chemical bond, pointing to a key role of the dopant. The molecule-like bimetallic cluster operates efficiently in both homogeneous and heterogeneous conditions, representing a special type of electrocatalyst. The molecule-like bimetallic cluster may thus provide a platform for the discovery of finely tuned catalysts, which could have broad implications for catalysis beyond H 2 production. Electrochemical methods SWV and LSV were conducted with an electrochemical workstation (model 660B; CH Instruments) in CH 2 Cl 2 (SWV) or THF (LSV) containing 0.1 M Bu 4 NPF 6 as a supporting electrolyte that was degassed and blanketed with a high-purity Ar gas. A GCE (3 mm diameter) was used as a working electrode, a Pt wire as the counter electrode and Ag/AgNO 3 (0.1 M AgNO 3 in CH 3 CN) as the reference electrode for the LSV experiments. SWV was carried out with a Pt disk (0.4 mm diameter) working electrode at 100 mV s −1 with a pulse height and a width of 20 mV and 20 ms, respectively. Ferrocene (Fc +/0 ) was added as an internal reference for Ag/AgNO 3 . Controlled potential electrolysis CPE experiments in homogeneous condition were conducted in a 5 ml cell containing 2.5 μM cluster and 1.0 M TFA dissolved in 2.0 ml THF (0.5 M Bu 4 NPF 6 ) that was degassed and blanketed with Ar gas. Electrolysis was conducted for 15 min under vigorous stirring with an electrochemical workstation (model 660B; CH Instruments) equipped with three electrodes consisting of glassy carbon plate working electrode (area=1 cm 2 ), a GDL (model N1S1007; CeTech Co., Taiwan) counter electrode (1 cm 2 ) and a Ag/AgNO 3 reference electrode. CPE experiments in heterogeneous condition were carried out for 60 min under vigorous stirring with a ZIVE MP1 potentiostat (WonATech, Korea) in an H-type cell that was equipped with a composite working electrode and a Ag/AgCl (3 M NaCl) reference electrode in one compartment and a platinum plate (1.68 cm 2 ) counter electrode in the other compartment. The working electrode was separated from the counter electrode by a proton exchange membrane (Nafion 117; Sigma-Aldrich). Both compartments were filled with 60 ml of 1.0 M Brinton–Robinson buffer (pH 3.0) that was degassed and blanketed with Ar gas. The composite working electrode was fabricated by spreading a catalyst ink prepared by mixing 16 μg of the cluster catalyst, 200 μg of carbon black (Vulcan XC-72) and 1.5 μl of Nafion solution (5 wt%; Sigma-Aldrich) in 50 μl of THF on a GDL (N1S1007; CeTech Co.) electrode (1 cm 2 ). For comparison, CPE experiments were conducted under the same condition using a commercial Pt/C (20 wt% platinum on Vulcan carbon black; Sigma-Aldrich) catalyst that was mixed with Nafion and dropcast on a GDL electrode (1 cm 2 ). The average size of Pt particle was 3.5±0.5 nm. The amount of H 2 evolved was quantified from an analysis of the headspace using an Agilent 7890B gas chromatography equipped with a thermal conductivity detector. Computational methods DFT calculations of the HER on Au 25 (SCH 3 ) 18 and PtAu 24 (SCH 3 ) 18 clusters were performed with the quantum chemistry program Turbomole V6.5. The def2-SV(P) basis sets were used for C, S and H, while effective core potentials which include scalar relativistic corrections and 19 (18) valence electrons were used for Au (Pt). Geometry optimization was done with the TPSS (Tao, Perdew, Staroverov and Scuseria) functional. In our calculations, solvent effects were treated implicitly by making use of the conductor-like screening model (COSMO) as implemented in Turbomole. Data availability The authors declare that all the other data supporting the findings of this study are available within the article and its Supplementary Information Files or from the corresponding author on reasonable request. How to cite this article: Kwak, K. et al . A molecule-like PtAu 24 (SC 6 H 13 ) 18 nanocluster as an electrocatalyst for hydrogen production. Nat. Commun. 8, 14723 doi: 10.1038/ncomms14723 (2017). Publisher’s note : Springer Nature remains neutral with regard to jurisdictional claims in published maps and institutional affiliations.